A two-atom electron pump With the development of single-atom transistors, consisting of single dopants, nanofabrication has reached an extreme level of miniaturization. Promising functionalities for future nanoelectronic devices are based on the possibility of coupling several of these dopants to each other. This already allowed to perform spectroscopy of the donor state by d.c. electrical transport. The next step, namely manipulating a single electron over two dopants, remains a challenge. Here we demonstrate electron pumping through two phosphorus donors in series implanted in a silicon nanowire. While quantized pumping is achieved in the low-frequency adiabatic regime, we observe remarkable features at higher frequency when the charge transfer is limited either by the tunnelling rates to the electrodes or between the two donors. The transitions between quantum states are modelled involving a Landau–Zener transition, allowing to reproduce in detail the characteristic signatures observed in the non-adiabatic regime. The first signatures of transport affected by a single dopant were obtained in microelectronics field-effect transistors [1] . Experiments on transport through a single-donor state followed thanks to a drastic downscaling of the gate length and a specific doping scheme [2] . Moreover, single-atom transistors were obtained with other techniques [3] , [4] , [5] , involving both random or deterministic placement of the dopant atoms. This rapid progress paved the way for electronics based on single dopants [6] , [7] , [8] . Interesting disruptive functionalities are expected when coupling several donor states and manipulating independently their charge or spin state. Such a two-atom transistor has been achieved recently, allowing to measure the spectrum of a single dopant by d.c. electrical transport [9] . Beyond d.c. transport, the next step consists in transfering a single electron over the two-coupled dopants in a controlled way, hence realizing an electron pump. Adiabatic charge pumping at zero d.c. bias, in contrast to stationary electronic transport at finite bias, results in a net direct current I =e f , when exactly one electron is transferred during a cycle of period 1/ f (refs 10 , 11 , 12 ). Electron pumping through many donors has been reported in a large structure [13] . Motivated by metrological applications [14] , there has been a growing interest in the non-adiabatic regime, where the modulation period is comparable to the characteristic time which particles spend in the system [15] , [16] , [17] , [18] . However, all experiments so far were carried out in either one of these regimes, but were not subsequently tuned to both. The ultra-scaled electron pump presented here, where we use real nanometre-size atomic orbitals instead of commonly used rather large dots, offers this unique opportunity. Here we demonstrate pumping of a single electron across two coupled donor states and investigate both the adiabatic and non-adiabatic regimes. Selection of coupled donor states We obtain transport through two dopants because we use three independent gates to control an extremely small volume of silicon (60 × 20 × 60 nm 3 ). The number of P dopants in this region is only a few tens, for a concentration of 10 18 cm −3 , below the metal–insulator transition ( Fig. 1 ). The parts of the wire uncovered by the gates and adjacent spacers are doped with arsenic donors at high concentration (≈10 21 cm −3 ) to define conducting source and drain electrodes, separated by 60 nm. This separation prevents transport through a single donor, which would require a much shorter structure [2] , but favours transport through two donors in series. Indeed, a distance of ≈30 nm between the two donors yields a mean tunnel coupling of the order of 1 GHz (ref. 19 ), a good compromise between weak coupling and measurable current. Moreover, we obtain separate control over the energy levels of the two dopants by splitting the top gate into two, which face each other at a distance of only 15 nm. Finally, a voltage V bg is applied to the substrate [9] to tune the coupling between the dopants and the leads and rule out rectification effects [20] , measured for instance in [21] . Starting from a nearly perfect yield in terms of transistor behaviour, the final yield for two-dopant features remains higher than 50% for the geometry and doping level chosen here. 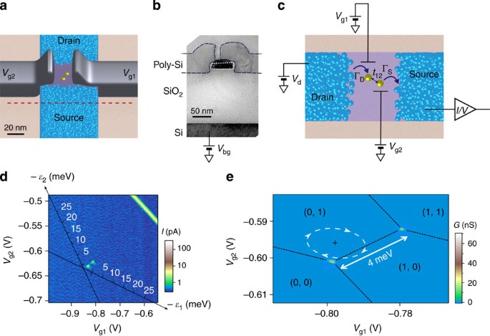Figure 1: Control of two dopants with three gates. (a) Schematic tilted view of the sample along the source–drain axis, with two phosphorus dopants in yellow in the small silicon region controlled by three gates. (b) Transmission electron micrograph of the cross-section of a nominally identical sample. The two top gates and the wire are highlighted by blue and white dashed lines, respectively. The cross-section is slightly offset from the gate region (along the red line ina), where the wire is thicker than below the gates because of the source/drain raised by epitaxy. The wafer substrate, separated by a 145-nm-thick SiO2layer, is used as a back gate. (c) Schematic top view of the sample including the gate and source–drain control parameters. (d) Source–drain current (I) withVd=2 mV,Vbg=11.5 V and superimposed axes giving the energy of each ionized donor with respect to the Fermi level in the leads. The two triangular triple points of the two-dopant system are isolated from any other visible single electron feature by at least 20 meV. (e) Triple points at small bias (Vd=50 μV) measured with a lock-in amplifier. The black dashed lines indicate regions of stable charge states (n1,n2), whereniis the number of electron on theith donor. The white dashed line shows an example of pumping trajectory realized inFig. 3c, around the working point indicated by the black cross. Figure 1: Control of two dopants with three gates. ( a ) Schematic tilted view of the sample along the source–drain axis, with two phosphorus dopants in yellow in the small silicon region controlled by three gates. ( b ) Transmission electron micrograph of the cross-section of a nominally identical sample. The two top gates and the wire are highlighted by blue and white dashed lines, respectively. The cross-section is slightly offset from the gate region (along the red line in a ), where the wire is thicker than below the gates because of the source/drain raised by epitaxy. The wafer substrate, separated by a 145-nm-thick SiO 2 layer, is used as a back gate. ( c ) Schematic top view of the sample including the gate and source–drain control parameters. ( d ) Source–drain current ( I ) with V d =2 mV, V bg =11.5 V and superimposed axes giving the energy of each ionized donor with respect to the Fermi level in the leads. The two triangular triple points of the two-dopant system are isolated from any other visible single electron feature by at least 20 meV. ( e ) Triple points at small bias ( V d =50 μV) measured with a lock-in amplifier. The black dashed lines indicate regions of stable charge states ( n 1 , n 2 ), where n i is the number of electron on the i th donor. The white dashed line shows an example of pumping trajectory realized in Fig. 3c , around the working point indicated by the black cross. Full size image The sample is measured at 150 mK in a dilution refrigerator. The source–drain current I is first measured with a fixed source–drain bias voltage V d to select two ideally placed dopants. The back gate voltage is changed until a set of triangles, characteristic of two levels in series [22] , is obtained when scanning the front gates ( Fig. 1d ). This coupled donor system allows to perform atomic spectroscopy, in contrast with a single-donor transistor based on the same technology where fluctuations of the local density of states dramatically affect the current at finite bias [23] . A large (10 meV) separation in energy between the ground and first excited states was measured in the same sample [9] as investigated here. Besides this large valley-orbit splitting that makes it quite insensitive to a small bias, our two-donor system is also well isolated in energy from any other states that could carry a current from source to drain ( Fig. 1d ). The two triple points are separated by a Coulomb repulsion energy E c =4.0±0.1 meV, which is markedly larger than any value reported so far [24] . Electron pumping To achieve pumping through two atoms, we set V d to zero and modulate the top gates ( i =1, 2) with phase-shifted sinewaves added to the d.c. voltages V g i = + sin(2π ft ± φ /2), to follow elliptical trajectories in the ( V g1 , V g2 ) plane possibly enclosing a triple point [11] ( Fig. 1e ). Adiabatic pumping occurs when the timescale of the driving is much larger than the timescale associated with tunnelling to the leads for an electron in the two-donor system, , and when there are no excitations in the internal dynamics due to the driving signal, requiring (see Equation 1). Here Γ is a tunnelling rate, δ ε = ε 1 − ε 2 the difference in energy between the two levels, the speed at which they cross, k B T the energy scale set by the temperature and t 12 the tunnel coupling between the two levels. Then the system follows the charge states given by the electrostatic stability diagram ( Fig. 1e ). 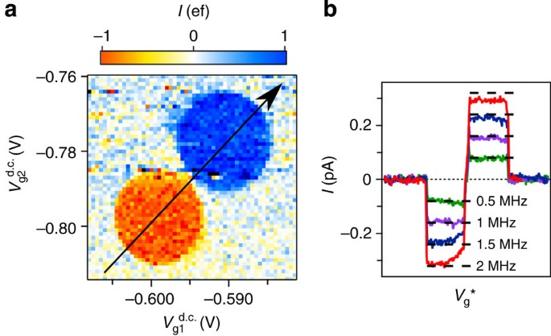Figure 2: Adiabatic electron pumping through the two dopants. (a) Map of the pumped current at 1 MHz and zero bias voltageVd. (b) Pumped current for different frequencies along thepath indicated by the arrow ina. Quantized pumpingI=±efis indicated by horizontal dashed lines. Figure 2 shows the normalized d.c. current I /e f measured in this regime. As expected we observe two circular regions of constant quantized current I =±e f , wherever a triple point is enclosed by the ellipse, and I =0 elsewhere. The sign of the current is reversed by changing the direction of the trajectory. The two-atom system offers intriguing advantages compared with other quantized electron pumps, due to the large energies at play in this system. The large Coulomb repulsion energy between the dopants ensures wide and flat plateaus for the pumped current versus V d : a slope of 1.9 GΩ is obtained over a V d range of 3.1 mV at 1 MHz ( Supplementary Fig. S1 ). In contrast with metallic Coulomb islands, co-tunnelling events via intermediate virtual states are strongly suppressed due to the 10 meV single-level spacing for each of the dopants [9] . Both these elastic co-tunnelling effects as well as remaining unwanted events due to inelastic tunnelling are shown to be small. Figure 2: Adiabatic electron pumping through the two dopants. ( a ) Map of the pumped current at 1 MHz and zero bias voltage V d . ( b ) Pumped current for different frequencies along the path indicated by the arrow in a . Quantized pumping I =± ef is indicated by horizontal dashed lines. Full size image At higher frequency the pumped current deviates from the fundamental relation I =e f . 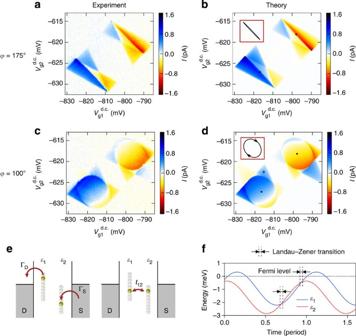Figure 3: Non-adiabatic electron pumping at 10 MHz. (a,c) Two-dimensional map of the current measured withφ=175°(a) andφ=100° (c) between the two driving signals as a function of the working point (,). (b,d) Simulation of the current with ΓD=670 MHz, ΓS=18 MHz andt12/h=610 MHz. The shape of the trajectory in the (Vg1,Vg2) plane is shown at the top left of the simulation for each phase difference (not to scale), and triple points are indicated with a dot. (e) Sketch of the model used for the previous simulation. Tunnelling to the leads occurs with rates ΓDand ΓS. Coupling between the two dopants by a tunnel amplitudet12leads to a Landau–Zener transition when the two levels cross each other. (f) Calculated energy levels as a function of time for the working point indicated by the black cross ind. Landau–Zener transitions occur as immediate events when the two levels cross (between the dashed lines). Figure 3a show the current map for f =10 MHz. The triple points are slightly shifted as compared to Figs 1 and 2 , because the sample was warmed up at room temperature in the meantime. The two circular regions appearing when enclosing the triple points are still visible in Fig. 3c , but the current inside is not independent of the working point anymore. This is the first manifestation of the deviation from the adiabatic regime. The second remarkable feature is the occurence of extra current outside these circular regions. This effect becomes dramatic in Fig. 3a , where, due to the vanishingly small surface area of the pumping cycle for φ =175°, no signal is expected in the adiabatic case. Figure 3: Non-adiabatic electron pumping at 10 MHz. ( a , c ) Two-dimensional map of the current measured with φ =175°( a ) and φ =100° ( c ) between the two driving signals as a function of the working point ( , ). ( b , d ) Simulation of the current with Γ D =670 MHz, Γ S =18 MHz and t 12 / h =610 MHz. The shape of the trajectory in the ( V g1 , V g2 ) plane is shown at the top left of the simulation for each phase difference (not to scale), and triple points are indicated with a dot. ( e ) Sketch of the model used for the previous simulation. Tunnelling to the leads occurs with rates Γ D and Γ S . Coupling between the two dopants by a tunnel amplitude t 12 leads to a Landau–Zener transition when the two levels cross each other. ( f ) Calculated energy levels as a function of time for the working point indicated by the black cross in d . Landau–Zener transitions occur as immediate events when the two levels cross (between the dashed lines). Full size image The complex features observed in the non-adiabatic regime can be fully understood by means of the model depicted in Fig. 3e and described in the Methods section. The transitions occuring within the two dopants are described through the dynamics of the closed two-level system. A dissipative part of the dynamics accounts for the tunnel coupling to the source and drain. The transition rates between donor states due to tunnelling to the leads are obtained from Fermi’s golden rule [25] and are proportional to the tunnelling rates to source and drain (Γ s and Γ D ). Hopping of an electron between the two dopants, with tunnel amplitude t 12 , can occur when the two levels cross each other and the resulting time evolution of the two-level system is described according to the Landau–Zener problem [26] . Consequently, the probability of staying on the same dopant after the crossing, that is, the transition from ground to excited state, is given by the Landau–Zener transition probability P LZ . Then the probability for an electron to move from one dopant to the other when the levels are aligned depends on the speed v and is given by, The strict separation of the dynamics of the closed system and of the coupling to the reservoirs is possible because the time during which the levels cross, ~2 t 12 / v , is of the order of 0.1 ns, and thus much smaller than the timescale related to the dissipative dynamics, . Using the electrostatic couplings obtained from the d.c. measurements, we reproduce the various features observed in the experiment with a unique set of parameters (Γ D =670 MHz, Γ S =18 MHz and t 12 / h =610 MHz ), as illustrated in Fig. 3b for φ =175° and φ =100°. The whole set of phase differences φ is simulated with the same fidelity ( Supplementary Movie S1 ). If non-adiabatic, the system does not necessarily relax to the ground state, either due to slow tunnelling to the leads or due to its internal dynamics ( P LZ differs significantly from zero, if the condition is no longer fulfilled). Each case yields characteristic features that we discuss in the following. We first focus on the working point indicated by the black cross in Fig. 3d . In this region no current is detected in the adiabatic regime. The time evolution of the energy levels is shown in Fig. 3f . Although the phase shift of the two driving voltages have a phase difference φ =100°, the energy level of the two dopants are phase shifted only by 44° due to the cross-talk between the gates and dopants, see Methods section for more details. Dopant 2 can accept electrons only from the drain and not from dopant 1, because it always lies below the Fermi level. After the electron moves to the dopant 1, its energy can be raised above the Fermi level, and it is eventually released into the drain lead. The key point here is that the transition probability between the two discrete dopant levels is different from one, otherwise the electron sitting on dopant 1 would go back to the initial dopant 2 after the second-level crossing. This missed tunnel event due to the Landau–Zener transition occuring with probability P LZ ≠0 in the non-adiabatic regime increases significantly the error rate [27] . Indeed, for this working point, we get P LZ ≈0.25 from the simulation for both crossings. In contrast, at low enough frequencies the electron always stays on the lowest energy level according to the adiabatic theorem ( P LZ ≈0). Also the rightmost red non-adiabatic feature can be understood in these terms. The non-adiabatic feature inside the circle is of different origin: here, it is the tunnelling dynamics that matters. Even though ε 2 is driven from above to below the Fermi energy before ε 1 , the slow tunnelling dynamics, 2π fv ~Γ 2 k B T , allows to charge dopant 1 first instead of 2. This effect is important in particular if the coupling between dopant 1 and the drain is much stronger than the coupling between dopant 2 and the source. Indeed, is fulfilled in the experiment, giving rise to the sign change within the circle. Note that this effect would survive even in the limit of P LZ ~0, hence it does not rely on a non-adiabatic level crossing. The additional features can be understood analogously and are influenced by the individual coupling strengths Γ S and Γ D , with the exception of one feature that will be discussed in the following. To reproduce the faint side triangle along the anti-diagonal, visible in Fig. 3d , we finally add a small effective inelastic relaxation rate Γ in =14 MHz between levels to the model. However, this rate has a very limited impact on the overall pumped current. For the working point indicated by the cross, the simulation shows that the total current signal is changed by only 10% due to this inelastic term, the remaining 90% being due to the elastic coupling t 12 . A much higher inelastic rate would suppress the current coming from the Landau–Zener transition. Importantly, the ultimate atomic size of the system is crucial to get large level separation and strong Coulomb interaction. This enables us to use driving amplitudes corresponding to an energy level modulation of ≈2.5 meV, much higher than the electronic temperature (300 mK) in the contact, ≈25 μeV. As a consequence the pumped current signal has remarkably sharp borders between different pumping regions, allowing a detailed study of the mechanisms at play in each of these regions. Moreover, due to the large amplitudes, interlevel transitions occur far away (with respect to k B T ) from the resonances with the leads, which justifies the zero temperature approach for our model. Finally, the crucial parameter determining the non-adiabaticity is the speed of the crossing, depending on the frequency as well as on the size of the ellipse. With the large amplitudes we use, the crossover to non-adiabaticity is significantly lowered towards lower frequencies making these effects easily accessible experimentally. In summary, we have demonstrated electron pumping in a two-atom transistor. A model taking into account the tunnel couplings to the leads and between the two donors energy levels reproduces all the specific features observed in the non-adiabatic regime. These results are extremely encouraging for future developments of dopant-based electronics, because our ultimate size system behaves like a nearly perfect two-level system. The full control of the well separated states in the dopants opens new opportunities for the study of pure spin pumping in a quantum system contacted to ferromagnetic leads [28] and for transporting quantum information [29] . Data simulation The simulation of the pumped charge separates into two types of evolution: the local dynamics and the coupling of the double-donor system to the external reservoirs. This is justified as the level crossing time, ~2 t 12 / v , is much shorter than the time evolution due to external coupling. In time intervals in which the difference of the two levels, ε 1 ( t )− ε 2 ( t ), is larger than the hopping t 12 , we use the master equation d P ( t )/d t = W ( t ) P ( t ) to describe the evolution due to coupling to external reservoirs. As the Coulomb interaction is large, different triple points have a large separation and we can treat their contributions separately, here focussing on the triple point involving one extra charge. Therefore, the vector P T =( P 0 , P 1 , P 2 ) contains the probabilities for either no excess charge on the dopants, P 0 , or one excess charge on dopant 1 or 2, P 1 or P 2 , respectively. The kernel W takes into account an inelastic contribution and coupling to the leads, where Θ( x <0)=0 and Θ( x ≥0)=1. It depends on the tunnelling rates to the leads, Γ S,D , the inelastic decay rate Γ in and on the position of the levels with respect to the Fermi level in the leads. Temperature smearing of the electronic distribution function in the leads is neglected, because the amplitudes of the level modulation are much larger than temperature. When the two levels cross, ε 1 ( t )= ε 2 ( t ), the dynamics of the double-donor system is computed via the coherent time evolution of the isolated system, resulting in the transition probability 1− P LZ ( P LZ being the Landau–Zener probability) for an exchange between the occupation of dopant i and j , P i ( t +Δ t )= P LZ P i ( t )+(1− P LZ )P j ( t ). This event is considered as immediate (Δ t →0 + ) because of the above-mentioned small level crossing time. The steady-state solution is obtained by imposing periodic boundary conditions, P ( t )= P (t+1/ f ), on the piece-wise evolution of P . The d.c. component of the current is obtained via the integral , with the current operator in vector form , and the charge of the electron e <0. The results obtained from this formula are plotted in Fig. 3b . Lever arm factors The relation between the chemical potential of the donors’ ground state and the gate voltages are described by the linear relation, Δ ε i =∑ j m ij Δ V g j . By measuring the double-donor system with a finite source–drain bias, we get triangular patterns from which we extract the matrix elements m ij as m 11 =0.150, m 12 =0.147, m 21 =0.072 and m 22 =0.303. We note that while dopant 1 is almost equally coupled to both gates, dopant 2 has a strong asymmetric couplings to the gates. This is enough to control independently each dopant. When two phase-shifted sinewaves are applied onto the gates, the corresponding chemical potentials get a different phase-shift due to the off-diagonal terms of m ij , i≠j . For instance, if we consider 90° shifted driving signals with 8.16 mV and 3.96 mV (corresponding to the actual gate amplitudes used in Fig. 3c in the main text), and , the corresponding chemical potentials’ evolution is and , and the actual phase shift of the levels is reduced from 90° to 38.5°. How to cite this article: Roche B. et al . A two-atom electron pump. Nat. Commun. 4:1581 doi: 10.1038/ncomms2544 (2013).